Large-scale DNA editing of retrotransposons accelerates mammalian genome evolution Retrotransposons had an important role in genome evolution, including the formation of new genes and promoters and the rewiring of gene networks. However, it is unclear how such a repertoire of functions emerged from a relatively limited number of source sequences. Here we show that DNA editing, an antiviral mechanism, accelerated the evolution of mammalian genomes by large-scale modification of their retrotransposon sequences. We find numerous pairs of retrotransposons containing long clusters of G-to-A mutations that cannot be attributed to random mutagenesis. These clusters, which we find across different mammalian genomes and retrotransposon families, are the hallmark of APOBEC3 activity, a potent antiretroviral protein family with cytidine deamination function. As DNA editing simultaneously generates a large number of mutations, each affected element begins its evolutionary trajectory from a unique starting point, thereby increasing the probability of developing a novel function. Our findings thus suggest a potential mechanism for retrotransposon domestication. Retrotransposons spread DNA fragments in different genomic contexts and thus have become major contributors to genomic innovation. As recently shown, many retrotransposons have 'exapted' to become exons, genes or promoters, or to acquire other novel functions [1] , [2] , [3] , [4] , [5] , [6] , [7] , [8] , [9] . To attain a new function, a retrotransposon must undergo a rare series of fortuitous mutations. However, when mutagenesis is serial, successful 'domestication' is expected to be prolonged. Retroviruses replicate through a single-stranded RNA intermediate, which is reverse transcribed and integrated into the host genome. Occasionally, multiple cytosine-to-uracil deaminations are introduced on the negative-strand retroviral DNA after reverse transcription by proteins of the APOBEC3 (apolipoprotein B mRNA-editing enzyme and catalytic polypeptide 3) family [10] , [11] , [12] , [13] . While encounter with APOBEC3 impairs some viruses, others successfully integrate into the host genome, bearing G-to-A mutations compared with their original sequence. This process is thus called DNA editing. In recent years, it was shown that active LTR (long terminal repeat) retrotransposons, which are endogenous retroviruses, can also be edited [14] , [15] , [16] , [17] , [18] , [19] , [20] , [21] . However, the impact of DNA editing on genome variability has not been explored to date [22] . Here, we show that DNA editing has been a frequent event in various genomes and retrotransposon families. As editing led to large-scale diversification of retrotransposons, it has potentially expedited their ability to gain new functions. Identification of editing sites To detect edited elements, we assumed that a newly edited element should be almost identical to its ancestral element except for a few dense clusters of G-to-A mismatches, as such clusters are the hallmark of APOBEC3 editing [10] , [11] , [12] , [13] . To confirm that the mismatches are due to DNA editing, we exploited the asymmetry, or strand specificity, of editing: as opposed to random mutagenesis, APOBEC3 generates C-to-U mutations specifically on the negative strand of the element (with respect to the ORF), yielding clusters of G-to-A mutations, but not C-to-T, on the positive strand [10] , [11] , [12] . We therefore aligned, pairwise, the positive strands of all retrotransposons from selected families, and scanned the alignments for windows containing a particularly large number of G-to-A mismatches but no mismatches of any other type ( Fig. 1 ). We estimated the probability of such extreme events based on the frequency of the other transitions (Methods). We considered as a product of 'editing' each element in which we found a cluster of G-to-A with sufficiently small probability (typically around 10 −10 ) and where the number of G-to-A mismatches in the cluster was greater than a certain minimal length (typically around 10). The parameter values were tuned to minimize the fraction of false positives, which we naturally defined based on the DNA-editing strand specificity. If the clusters we observed were due to random mutagenesis and not to editing, we would expect to see a similar number of G-to-A and C-to-T clusters. Therefore, a greater number of G-to-A clusters compared with the number of C-to-T clusters indicates a low false-positive rate, and that the observed mutations are mostly the result of editing. 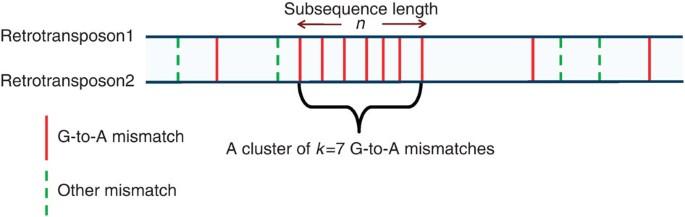Figure 1: A schematic representation of the computational method. The drawing shows a hypothetical alignment between two retrotransposons that has several mismatches, most of which are G-to-A. To detect editing, we scan the alignments for long clusters of G-to-A mismatches not separated by any other mismatch. We then calculate the probability that such a cluster (havingkG-to-A mismatches over a subsequence of lengthn) occurred by chance, based on the probabilities of C-to-T and T-to-C transitions (Methods). Figure 1: A schematic representation of the computational method. The drawing shows a hypothetical alignment between two retrotransposons that has several mismatches, most of which are G-to-A. To detect editing, we scan the alignments for long clusters of G-to-A mismatches not separated by any other mismatch. We then calculate the probability that such a cluster (having k G-to-A mismatches over a subsequence of length n ) occurred by chance, based on the probabilities of C-to-T and T-to-C transitions (Methods). Full size image DNA editing in mouse The mouse retrotransposons intracisternal A-particle (IAP) and early transposon (ETn/MusD) were edited when transfected into HeLa cells together with APOBEC3G [16] , and some of their genomic elements were found to be edited relative to their consensus [16] . We scanned the pairwise alignments of the entire IAP family for stretches of at least 12 consecutive G-to-A mismatches that occurred by chance with probability at most 10 −12 , based on the frequency of the other transition mutations (Methods). Strikingly, even with these very stringent thresholds, we identified a high level of editing: 195 IAP elements had large clusters of G-to-A mismatches containing 3,539 edited nucleotides ( Table 1 ; Fig. 2a ; Supplementary Data 1 , and Supplementary Figs S1-S4 ). Editing in these sequences is highly significant: our cutoffs were so stringent that not even a single C-to-T cluster was observed. The actual number of edited elements is probably much higher, as relaxing the thresholds up to a false-positive rate (number of C-to-T clusters/number of G-to-A clusters; Methods) of about 10% yielded 446 edited elements and 7,144 edited nucleotides ( Table 1 ; Fig. 2b,c ). Investigation of the sequences surrounding the edited nucleotides revealed dominance of adenosines at position +2 relative to the editing site ( G xA→ A xA motif; the underlined G is the editing site; Methods and Supplementary Table S1 ). This is in agreement with previous experimental studies [14] , [15] , [16] , [17] , [18] , [19] , [20] , [23] , [24] and supports the identification of these mismatches as an outcome of mouse APOBEC3 activity. Table 1 The number of edited elements identified in this study. 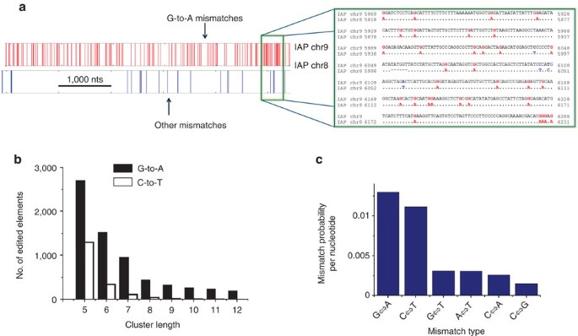Figure 2: Editing in mouse IAP. (a) An example of DNA editing. The IAP element at chr8:28575443-28581824 (build 37; 6,382 nts) aligns to the element at chr9:114987516-114993954 with 176 G-to-A mismatches and only 26 other mismatches. The G-to-A mismatches are plotted in the top left panel as bars at the coordinates where they occur. The lower left panel shows the much lower number of all other mismatches. The box on the right shows the actual alignment for a segment of 420 nts. The segment contains 32 G-to-A mismatches (red) and only 4 other mismatches (blue). (b) The number of edited IAP elements plotted against the cluster length. The number of elements that contain a C-to-T cluster is plotted as a control. The larger the cluster size we demand, the fewer elements we find, but the higher the confidence that these mismatches occurred because of editing. The thresholdP-value for recognizing the cluster as edited was set for convenience as 10−cluster length(Methods). (c) The probabilities of the individual pairs of mismatches across the entire IAP family. The mismatches G⇔A (that is, G-to-A and A-to-G) and C⇔T (C-to-T and T-to-C) are overrepresented, as expected, with a small excess of G⇔A. Mismatches were recorded along all aligned pairs of IAP elements. Full size table Figure 2: Editing in mouse IAP. ( a ) An example of DNA editing. The IAP element at chr8:28575443-28581824 (build 37; 6,382 nts) aligns to the element at chr9:114987516-114993954 with 176 G-to-A mismatches and only 26 other mismatches. The G-to-A mismatches are plotted in the top left panel as bars at the coordinates where they occur. The lower left panel shows the much lower number of all other mismatches. The box on the right shows the actual alignment for a segment of 420 nts. The segment contains 32 G-to-A mismatches (red) and only 4 other mismatches (blue). ( b ) The number of edited IAP elements plotted against the cluster length. The number of elements that contain a C-to-T cluster is plotted as a control. The larger the cluster size we demand, the fewer elements we find, but the higher the confidence that these mismatches occurred because of editing. The threshold P -value for recognizing the cluster as edited was set for convenience as 10 −cluster length (Methods). ( c ) The probabilities of the individual pairs of mismatches across the entire IAP family. The mismatches G ⇔ A (that is, G-to-A and A-to-G) and C ⇔ T (C-to-T and T-to-C) are overrepresented, as expected, with a small excess of G ⇔ A. Mismatches were recorded along all aligned pairs of IAP elements. Full size image Further analysis of the edited elements showed that the IAP subfamily most edited is IAPEz-int ( Supplementary Table S2 ). 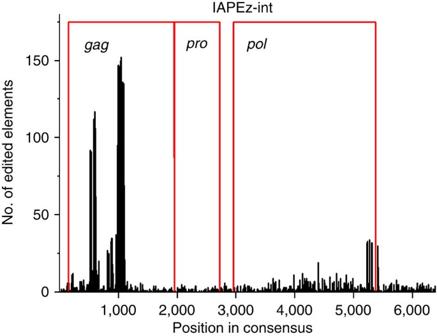Figure 3: Localization of the editing sites in the IAP sequence. We aligned each edited element from the IAPEz-int subfamily to the subfamily consensus. We then identified the position on the consensus sequence of each edited nucleotide, and created a histogram of the number of elements that were edited at each position along the consensus (Methods). The three open-reading frames of the element are indicated as red boxes. The locations of the edited nucleotides on the consensus sequence of this subfamily are shown in Figure 3 (Methods). Editing was found in 851 nucleotides out of the 6,388 of the retrotransposon. The pol ORF is less edited: 0.84 elements are edited, on average, at each potentially edited nucleotide at the pol region, compared with 3.25 in the other ORFs ( P <0.07; Mann–Whitney U (MWU) test). The third position of each codon is more (but not significantly) edited, with editing in 2.54 elements on average, compared with 2.07 and 1.87 in the first and second positions, respectively. There are 33 tryptophan codons (TGG) in the consensus sequence; 21 of them are edited in at least one element, which could lead to the creation of a stop codon. Figure 3: Localization of the editing sites in the IAP sequence. We aligned each edited element from the IAPEz-int subfamily to the subfamily consensus. We then identified the position on the consensus sequence of each edited nucleotide, and created a histogram of the number of elements that were edited at each position along the consensus (Methods). The three open-reading frames of the element are indicated as red boxes. Full size image Scanning pairwise alignments of MusD elements revealed, as expected, editing level and motif similar to that of IAP ( Table 1 ; Supplementary Table S1 and Supplementary Fig. S5 ). We also analysed the long interspersed nuclear elements (LINE) family of mouse retrotransposons (specifically, L1 elements). Our screen detected over 6,000 edited L1 elements (0.74% of the total number of L1 elements in the mouse genome; Table 1 ; Supplementary Fig. S6 ). The absence of editing in a previous screen of mouse L1 elements [16] could either be due to the very small number of elements screened or because clusters were not looked for. DNA editing in primates and other mammalians In primates, as in rodents, retrotransposons occupy nearly half of the genome, including some recently, or even currently, active elements [2] . The APOBEC3 gene family expanded in primates and underwent particularly strong positive selection [24] , [25] , [26] . We thus expected to find that editing has had a significant role also in primate genome evolution. We applied our method to several human endogenous retro virus (HERV) elements, including HERV-K, a retrotransposon family that was shown to be recently active [27] , [28] , [29] , [30] , and found editing in hundreds of elements in both human and chimpanzee (mostly in HERV-K and HERV-9; Table 1 ; Supplementary Table S2 and Supplementary Fig. S7 ). In human LINEs, more than a thousand additional edited elements were identified ( Table 1 ). However, the percentage of edited LINE elements is relatively small ( ∼ 0.1%), consistent with the low mutation rate of L1s even when experimentally inhibited by APOBEC3 [31] , [32] , [33] . The most edited families were L1PA2, L1PA3, L1PA5 and L1PA6 (ref. 34 ) ( Supplementary Table S2 ; Supplementary Fig. S8 for the locations of the edited nucleotides along the sequence of L1PA6). Human editing sites did not show sequence preference, perhaps because the observed sites are due to the combined action of a number of APOBEC proteins, or other proteins yet to be identified. We also screened the genomes of other mammals and found evidence for DNA editing in LTR elements of rat, marmoset, orangutan and rhesus ( Supplementary Table S3 ), suggesting that DNA editing is common across many mammalian species. As a negative control, we observed no or low traces of editing in the genomes of several non-mammalian species that contain retrotransposons but no APOBEC3 (ref. 35 ) (for example, chicken, yeast, worm and others; Supplementary Table S4 ). Expression and possible function of edited elements Extensively edited elements have probably lost their capacity to independently replicate. Nevertheless, we found edited elements that are expressed. In IAP, 35 edited elements (from our set of 446 low confidence edited IAPs; Supplementary Data 1 ) overlap with an exon (8%; Methods), more than in unedited IAP elements (904/26,508; 3.5%; P -value <10 −5 ; binomial test). Exonization of retrotransposons is known to contribute to alternative splicing [36] . Indeed, we found that the exon overlapping with many edited IAP elements is alternatively spliced (23/35 cases (66%); Supplementary Data 1 ). This amount of alternative splicing is greater than for unedited IAP elements (231/904; 26%; P <10 −6 ; binomial test). Although expression and alternative splicing do not directly imply function, these results might hint on a larger exaptation potential of the edited elements. A few expressed edited elements also overlap with reference genes. For example, the last exon of the mouse gene AK036462 overlaps with the edited IAP element at chr5:138302833-138303063 (build 37), with editing 50 nts downstream the 3′-splice site ( Fig. 4a ). Similarly, the fourth exon of the mouse gene AK132687 overlaps with the edited LINE element at chr12:92073349-92079863 ( Fig. 4b ). Here, editing modified the nucleotide at position −2 of the 5′-splice site. In both cases, the exons are supported by several spliced expressed sequence tags (ESTs), and as expected, the genes are mouse-specific. In human, the human-specific exon of the SLC22A20 transporter gene overlaps with the edited SVA (SINE-R, VNTR and Alu) element at chr11:64762642-64764372 (build 36; Fig. 4c ; see below on SVA) [37] , [38] . In this gene, editing introduced an adenosine at the nucleotide upstream of the 5′-splice site, modifying the 5′-splice site from the consensus G|GT [39] to A|GT (| indicates the exon–intron boundary). Editing could thus have contributed to the weakening of the 5′-splice site. Indeed, in the alternative known form of the gene, this exon is skipped. 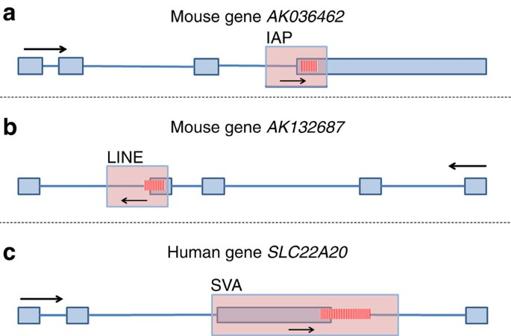Figure 4: Examples of editing in mouse and human genes. Three genes whose exons overlap with an edited element (from (a) the low confidence set, or (b,c) the high confidence set). (a) The truncated IAP element at chr5:138302833-138303063 (231 nts) aligns to chr10:24713242-24713464 with 26 mismatches, out of which 12 are G-to-A. It overlaps with the mouse geneAK036462. (b) The (full-length) LINE element at chr12:92073349-92079863 (6515 nts) aligns to chr6:104329142-104335592 with 40 mismatches, out of which 17 are G-to-A. It overlaps with the mouse geneAK132687. (c) The human (full-length) SVA element at chr11:64762642-64764372 (1731 nts) aligns to chr20:56422605-56423568 with 73 mismatches, out of which 35 are G-to-A. It overlaps with the human geneSLC22A20. Filled light-blue rectangles indicate exons and lines represent introns. The edited elements are denoted as large transparent pink boxes and the red stripes correspond to edited nucleotides. Arrows indicate the direction of transcription of the genes and the retrotransposons. The drawing is not to scale. Figure 4: Examples of editing in mouse and human genes. Three genes whose exons overlap with an edited element (from ( a ) the low confidence set, or ( b , c ) the high confidence set). ( a ) The truncated IAP element at chr5:138302833-138303063 (231 nts) aligns to chr10:24713242-24713464 with 26 mismatches, out of which 12 are G-to-A. It overlaps with the mouse gene AK036462 . ( b ) The (full-length) LINE element at chr12:92073349-92079863 (6515 nts) aligns to chr6:104329142-104335592 with 40 mismatches, out of which 17 are G-to-A. It overlaps with the mouse gene AK132687 . ( c ) The human (full-length) SVA element at chr11:64762642-64764372 (1731 nts) aligns to chr20:56422605-56423568 with 73 mismatches, out of which 35 are G-to-A. It overlaps with the human gene SLC22A20 . Filled light-blue rectangles indicate exons and lines represent introns. The edited elements are denoted as large transparent pink boxes and the red stripes correspond to edited nucleotides. Arrows indicate the direction of transcription of the genes and the retrotransposons. The drawing is not to scale. Full size image DNA editing is likely ongoing To determine whether DNA editing is also involved in recent retrotransposition events, we examined human SVA elements, which are hominoid-specific and are thus relatively new [40] , [41] . As far as we know, SVAs have not yet shown to be affected by APOBECs. We detected, with high confidence, 690 edited SVA elements (20.1% of all SVAs, the highest ratio in this study; Table 1 ; Supplementary Fig. S9 ). This set includes 238 human-specific elements and 16 polymorphic elements (out of the 77 polymorphic SVAs found in dbRIP [42] (database of polymorphic retrotransposons); Supplementary Data 1 ), demonstrating that DNA editing is an ongoing process. Chimpanzee SVA elements [43] were also edited, but with less confidence (about 20% false-positive level of C-to-T clusters); the recently active chimpanzee-PtERV elements [44] were edited with high confidence ( Table 1 ). In about 30 cases, the source of the SVA element was previously identified by locating the origin of its 5′-transduced sequence [37] . Fourteen of those elements were detected as edited according to our screen, but only when aligned to elements different from their predicted sources. This could indicate that editing of some of the sites we observed in SVA did not occur during the most recent retrotransposition event. These editing sites might reflect a more complicated, yet to be determined, historic chain of editing and retrotransposition events. The mechanism by which genomic repetitive elements evolved to gain various novel functions is one of the most intriguing questions in evolution. As editing modifies a large number of nucleotides simultaneously, it can change a given element to such an extent that subsequent random mutagenesis could lead to a different evolutionary trajectory compared with the original element, without having to cross valleys of low fitness [45] . Therefore, DNA editing can explain how some retrotransposons have acquired such a diverse collection of functions. Indeed, accelerated evolution due to editing has been demonstrated in the exogenous HIV virus, in which editing can result in drug resistance [46] . Another consequence of our results arises in the field of phylogenetics. Traditionally, the number of mismatches between two homologous sequences is an estimate of the time since their divergence (molecular clock). Large-scale editing greatly accelerates the rate of mutagenesis [47] , and thus can give the impression that edited retrotransposons are much older than they really are. Thus, editing must be taken into account when generating phylogenetic trees. This could be implemented, for example, by masking G-to-A mismatches between edited elements and their sources, or between all pairs ( Supplementary Fig. S10 ). Additionally, knowledge of DNA editing can assist in reconstructing the chronology of retrotransposition events, as an edited element (the one that has As in the G-to-A mismatch cluster) is less likely to precede its source element (the one with Gs; Supplementary Fig. S11 ). We applied our method also to a few human SINE elements and pseudogenes, as they too replicate through an RNA intermediate and reverse transcription. However, we did not find evidence for editing in these elements. We cannot rule out the possibility that some of these elements actually were edited: for example, it could be that editing affected some other SINE elements that we did not screen. Even for the retrotransposons that we screened, it could be that we were missing many edited elements because our screen was not sensitive enough or because the edited retrotransposons diverged too widely for editing to be detected. This is consistent with our finding of relatively high level of editing in the more recent hominoid-specific SVAs. In general, our method restricts the false-positive rate (because of the strand specificity property), but the false-negative rate can be quite high. Therefore, the full scope of editing is yet to be discovered. Databases All genomic data were extracted from the UCSC Genome Browser tables ( http://genome.ucsc.edu ) [48] . Mouse assembly was from July 2007 (mm9), human and chimpanzee from March 2006 (hg18 and panTro2, respectively). Retrotransposons were extracted from the RepeatMasker track ( http://www.repeatmasker.org/ ) of the UCSC genome browser. In mouse, IAP sequences were obtained by filtering for repeat names with *IAP*; filtering for *ET* gave MusD sequences. LINE1 elements were found by searching for repeat family L1, and rat ERV elements by searching for families with *ERV*. Primate HERV elements were extracted by filtering for repeat names with *HERV* (excluding the HERVH*subfamily). Human SVA elements were found by searching for repeat names *SVA*. Chimpanzee PtERV were found by filtering for repeat names PtERV*. Editing detection algorithm To detect editing, we divided all retrotransposons under consideration to subfamilies (based on the RepeatMasker annotation) and aligned all elements of the same subfamily, pairwise (not to the consensus), using NCBI BLASTn ( http://www.ncbi.nlm.nih.gov/blast ) [49] . We used a small E -value of 10 −50 to guarantee that we compare only highly similar elements that differ by just a few mutations. We disabled the low complexity filter and otherwise used the default BLAST parameters. We characterized DNA-editing events as alignments with an exceedingly high density of G-to-A mismatches, which could not be explained as a random accumulation of mutations. To find these G-to-A clusters, we searched for subsequences in which the number of G-to-A mismatches in the alignment was exceedingly high. To assess the significance of a cluster of k G-to-A mismatches in a subsequence of length n , we first recorded the number C-to-T and T-to-C mismatches in the aligned pair to approximate the probability of a transition mutation per nucleotide: Under the null hypothesis of no editing and assuming symmetry between all transitions and that transversions are negligible (see Fig. 2 ), the probability to find at least k G-to-A mismatches in a subsequence of length n is given by the binomial distribution: For n >20 and P <0.05, we used the Poisson approximation to the binomial distribution. For each alignment, we systematically searched for the maximal subsequence containing at least k min G-to-A mismatches in which P is less than a threshold P max . A schematic representation of a G-to-A mismatch cluster is plotted in Figure 1 . According to equation (2), the cluster of G-to-A mismatches could or could not be interrupted by other mismatches. We did not observe any qualitative difference in the results when the G-to-A mismatches were not forced to be consecutive. Nevertheless, to increase confidence, for all the results reported in the main text, the G-to-A mismatches were consecutive. Occasionally, multiple edited subsequences were identified for a given alignment, as long as each edited subsequence satisfied k ≥ k min and P < P max . In addition, elements were frequently found to be involved in editing when compared with more than one other sequence. In Table 1 , we report the number of unique edited nucleotides and elements in each retrotransposon subfamily. Because of the large number of pairwise alignments, it is expected to find some significant clusters just by chance. We accounted for these false positives directly, by taking advantage of the strand specificity. If the clusters of the G-to-A mutations were purely due to chance, we would expect to see a similar number of significant C-to-T (or T-to-C) clusters. However, editing replaces C by U in the (−) strand of the single-stranded DNA of the element, inducing a G-to-A mutation in the (+) strand. Therefore, editing is strand-specific and is expected to yield only G-to-A clusters of mismatches. We thus repeated the search for clusters, but with the role of A-to-G and C-to-T reversed, that is, we looked for clusters of C-to-T, while calculating p (the probability of a transition, equation (1)) from the number of A-to-G and G-to-A mismatches. We approximated the number of false-positive G-to-A edited elements as the number of elements with C-to-T 'editing' (see also Supplementary Fig. S12 ). We ran this procedure for several values of P max and k min until we reached the desired level of false-positive rate (either zero or almost zero for the high confidence set, or about 10% for the low confidence set). The final values of the parameters ranged between 10 −15 –10 −6 for P max and 5–12 for k min and are given in Supplementary Table S5 . Identifying the locations of the edited nucleotides We downloaded the consensus sequences of the retrotransposon subfamilies (mouse) IAPEz-int and (human) L1PA6 from Repbase ( http://www.girinst.org/repbase/ ). These subfamilies were most edited in their respective families. We then aligned each edited element from these subfamilies (from the low-confidence set as described in Table 1 ) to the subfamily consensus using BLAST (blastn, E -value 10 −50 , no filtering). We considered only the top-ranked alignment for each element. Using the alignments, we mapped the location of each edited nucleotide into the consensus sequence, and created a histogram of the number of elements edited at each nucleotide of the consensus. We removed editing sites in which the consensus was not A or G. The ORFs in the consensus sequences were located using ORF finder ( http://www.ncbi.nlm.nih.gov/gorf/ ). Coordinates of edited elements and nucleotides The coordinates of all edited elements and nucleotides described in this study are listed in Supplementary Data 2 . Identifying motifs We searched for a motif in each edited element separately. We first calculated the frequencies of A, C, G, and T nucleotides separately in each retrotransposon subfamily. Then, for each edited element, we looked at all nucleotides at a given position with respect to the mismatch sites. Consider a cluster of k mismatches, m out of which share the same nucleotide at a given position with respect to the mismatch. The probability for an event as rare as this to happen by chance is given by the binomial distribution (as in equation (2)). Here, p is the relative frequency of the nucleotide in the retrotransposon subfamily, taken from the pre-processing step. The equation for the P -value is: An element is considered to have a motif at a given position if the P -value is less than a given threshold. Analysis of expression In the IAP expression analysis, we compared the low-confidence edited elements ( Table 1 ) to all other IAP elements. We uploaded the coordinates of the edited elements to the UCSC genome browser and calculated the number of elements that overlap with an exon (the UCSC mRNA track). The P -value for the expression of edited elements was calculated using a binomial test, with the probability of an element to be expressed taken from the non-edited elements. To detect alternative splicing, we first created a UCSC track with the base-pair wise intersection of the edited elements and the exons. We then intersected this track with all introns (again obtained from the mRNA track) and merged adjacent intervals. We report the total number of these intervals, which represent edited IAP elements that have an overlap with both an exon and an intron. We repeated the calculation for the non-edited elements, and calculated the P -value as above. How to cite this article: Carmi, S. et al . Large-scale DNA editing of retrotransposons accelerates mammalian genome evolution. Nat. Commun. 2:519 doi: 10.1038/ncomms1525 (2011).